Single-photon-level quantum image memory based on cold atomic ensembles A quantum memory is a key component for quantum networks, which will enable the distribution of quantum information. Its successful development requires storage of single-photon light. Encoding photons with spatial shape through higher-dimensional states significantly increases their information-carrying capability and network capacity. However, constructing such quantum memories is challenging. Here we report the first experimental realization of a true single-photon-carrying orbital angular momentum stored via electromagnetically induced transparency in a cold atomic ensemble. Our experiments show that the non-classical pair correlation between trigger photon and retrieved photon is retained, and the spatial structure of input and retrieved photons exhibits strong similarity. More importantly, we demonstrate that single-photon coherence is preserved during storage. The ability to store spatial structure at the single-photon level opens the possibility for high-dimensional quantum memories. Light with orbital angular momentum (OAM) has many exciting applications, including optical communications [1] , [2] , trapping of particles [3] , [4] and astrophysics [5] , [6] . In quantum information and quantum optics, light has been encoded with information in its OAM degrees of freedom [7] , [8] , enabling networks to carry significantly more information and considerably increase their capacity. Moreover, these higher-dimensional states enable more efficient quantum-information processing, and the large-alphabet quantum key distribution affords a more secure flux of information [9] . Establishing a quantum network involves the coherent interaction [10] between light and matter. There are already some experiments based on such light-matter interfaces—for example, establishing OAM entanglement of a photon and collective atomic-spin excitations [11] , [12] and storing light in matter [13] , [14] , [15] , [16] , [17] , [18] , [19] , [20] , [21] . Recently, light carrying OAM or a spatial structure has been stored via electromagnetically induced transparency (EIT) in an atomic ensemble [13] , [14] , [15] , [16] , in a cryogenically cooled doped crystal [17] , via gradient echo technique in an atomic ensemble [18] , [19] , [20] , and using atomic frequency comb techniques in solids doped with rare-earth-metal ions [21] . However, these important works involve bright sources. Very recently, work has begun on storing such light at near single-photon levels [22] , [23] ; however, still this light is a strongly attenuated laser, not a true single photon. So far, there is no report on imaging at a true single-photon level. In quantum information science, the reversible transfer of a quantum state between a true single photon and matter is essential, as it is a crucial resource in operating quantum repeaters, having the potential to overcome distance limitations of quantum communication schemes through transmission losses. Grodecka et al . [24] show theoretically that the transverse as well as longitudinal degrees of freedom constitute a valuable resource for multimode quantum memories with excellent capacities. Here we report the first experimental realization of a multimode optical memory at true single-photon levels via EIT. In our experiment, we prepare non-classical correlated photon pairs using spontaneous four-wave mixing (SFWM) via a double-lambda configuration in a cold 85 Rb atomic ensemble. One photon of each pair is used as a trigger; the other is mapped and stored in a second cold atomic ensemble via EIT. Each photon to be stored carries one OAM unit per photon (in units of ). After a programmed storage time, the photon can be retrieved. We not only prove experimentally that the non-classical correlation between the trigger photon and the retrieved photon is maintained but also demonstrate that the spatial structure of the photon is also very well preserved during storage. More importantly, we show with the aid of a Sagnac interferometer that coherence of the single photon is also preserved. Our results show that this approach is promising for realizing a high-dimensional quantum memory in the future. Preparing a true single photon The single photon used in the experiment was prepared using SFWM in a cold 85 Rb atomic ensemble trapped in a two-dimensional magneto-optical trap (MOT) [25] . In the simplified experimental setup in Fig. 1(a) , photon signal 1 at 780 nm is used as a trigger and photon signal 2 at 795 nm is stored for subsequent treatment; therefore, we hereafter call photon signal 1 the trigger and photon signal 2 the signal. We first proved the existence of a non-classical correlation between these two photons by demonstrating a strong violation of the Cauchy–Schwarz inequality [26] . Furthermore, we also demonstrated the single-photon property of the signal photon by performing the Hanbury–Brown and Twiss (HBT) experiment on the trigger photon [27] , [28] . Experimentally, we obtained an α value of 0.025±0.005 for the signal photon. For an ideally prepared single-photon state, the anticorrelation parameter α goes to zero [27] , [28] . Details of the experiment are presented in the Methods. 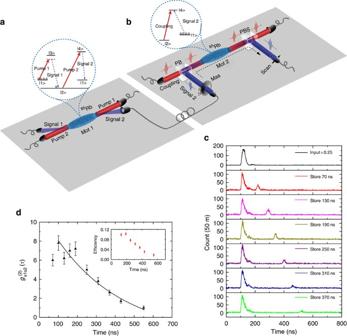Figure 1: Storage of a single photon. (a) Simplified diagram depicting the generation of non-classical photon correlations using SFWM. MOT: magneto-optical trap. Inset: energy level diagram for SFWM (see Methods). (b) Photon storage diagram. PBS: Glan–Taylor polarization beam splitter with the extinction ratio of 105:1. Inset: energy level diagram for EIT (see Methods). (c) Coincidence counts between the retrieved signal and the trigger as a function of storage time. (d) Cross-correlation functiongs1,s2(τ) between the retrieved signal and the trigger photons against the storage time. The solid line is the exponential fitAe−τ/T+g0tog(2)s1s2(τ) (whereA=13.3,T=348,g0=−1.89). The inset shows the efficiency function against storage time. All data are raw, without noise correction. Error bars represent±one standard deviation and are calculated based on the count statistics of single photons. Figure 1: Storage of a single photon. ( a ) Simplified diagram depicting the generation of non-classical photon correlations using SFWM. MOT: magneto-optical trap. Inset: energy level diagram for SFWM (see Methods). ( b ) Photon storage diagram. PBS: Glan–Taylor polarization beam splitter with the extinction ratio of 10 5 :1. Inset: energy level diagram for EIT (see Methods). ( c ) Coincidence counts between the retrieved signal and the trigger as a function of storage time. ( d ) Cross-correlation function g s1,s2 ( τ ) between the retrieved signal and the trigger photons against the storage time. The solid line is the exponential fit A e − τ / T + g 0 to g (2) s1s2 ( τ ) (where A =13.3, T =348, g 0 =−1.89). The inset shows the efficiency function against storage time. All data are raw, without noise correction. Error bars represent±one standard deviation and are calculated based on the count statistics of single photons. Full size image We next stored single photons not carrying any spatial structure via EIT in the second atomic ensemble (see Fig. 1b ). Cross-coincidence counts were measured between the trigger photon and the leaked signal photon and the retrieved signal photon ( Fig. 1c ). We also measured the efficiency of storage against storage time ( Fig. 1d ). The inset shows the efficiency as a function of storage time; the maximum efficiency obtained was ~10%. We find that even after about 400 ns of storage, a strong non-classical correlation between the retrieved signal photon and the trigger photon still persists. Details of the experiment are also given in the Methods. Furthermore, we checked the single-photon nature of the signal photon after storage again by performing the HBT experiment with the trigger photon [27] , [28] . An α value of 0.32±0.08 was obtained for the retrieved signal photon having been stored for about 190 ns, confirming clearly that the single-photon nature is preserved during storage. In our experiment, α changed from 0.025 (before storage) to 0.32 (after storage); we estimated that the noise from the scattering of coupling contributed about 0.16 to α . More strict filtering could reduce this kind of noise further. The remaining contribution to α was mainly from the attenuation of the single photon during the storage, retrieval and the measurement. The noise generated through delayed four-wave mixing process could be negligible because of the large detuning of 3 GHz in our experimental energy level configuration and the small optical depth (OD) of the memory [29] in our system. In the HBT measurement, the detection system registers the particle-like property of the state irrespective of losses. For an ideal single photon, it cannot be divided into two parts and detected by two different detectors simultaneously; therefore, α goes to zero for a near perfect single photon state. The criterion shown in Filip et al . [30] shows that even for a state expressed as ρ = P |0><0|+(1− P )|1><1|, with P >0.5, where P is the probability of the vacuum state caused by all losses of the single photon before it reaches the detection system (in our experiment, 1− P corresponds to the storage efficiency), which has a positive Wigner function, but it cannot be expressed as a mixture of Gaussian states, is still a non-classical state. Storing a single-photon-carrying OAM To store a single-photon-carrying spatial structure, we inserted a spiral phase plate (VPP-1c, RPC Photonics, transmission coefficient >95%) in the optical path along which the signal photon is transmitted. The signal photon now carried a donut-shaped structure (see the CCD camera image in Fig. 2a taken after the light beam has traversed the plate; the power-distribution curve along the transverse direction is given above); this signal has a well-defined OAM of 1 . After ~100 ns in storage in MOT 2, the signal photon was retrieved and collected into a single-mode fibre; the tip of the fibre was scanned along the transverse direction. Before performing the storage experiment, we balanced the coupling efficiency of the fibre at different points along the transverse direction. During the experiment, we initially scanned the transverse position of the tip of the receiver fibre and measured the cross-correlation function between the input signal and the trigger photons, obtaining a donut-shaped curve, as shown in Fig. 2b ; see also Fig. 2a . 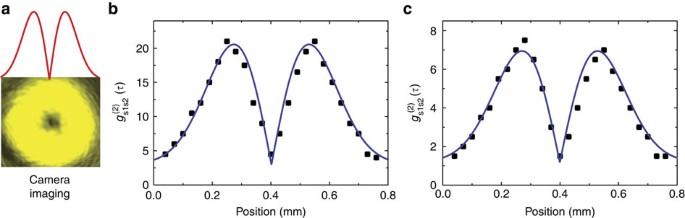Figure 2: Storage of a true single photon carrying an OAM. (a) Image of a laser beam after traversing the spiral phase plate. The red line is the power-distribution curve along the transverse direction. (b) Cross-correlation between input signal and trigger photons, obtained by scanning the transverse position of the input signal; (c) cross-correlation function between retrieved signal and the trigger photons. The solid lines in (b) and (c) are theoretical fits. All data are raw, without noise. Figure 2c shows the cross-correlation function, also donut-shaped, between the retrieved signal and the trigger photons. To compare Fig. 2b,c , we calculated image visibility and similarity. The former is obtained from , where g s1,s2,max ( g s1,s2,min ) are the maximal (minimal) cross-correlation values, which were 0.9 and 0.88 for the retrieved signal and for the input signal, respectively. We also analysed the fidelity of the retrieved image by calculating the similarity , where A and B are the grey-scale matrices of the two images to be compared [20] . High similarity means high fidelity. The calculated similarity of the retrieved image was 0.996. In our calculation, m is fixed because we only scanned the tip of the fibre along the transverse direction. Figure 2: Storage of a true single photon carrying an OAM. ( a ) Image of a laser beam after traversing the spiral phase plate. The red line is the power-distribution curve along the transverse direction. ( b ) Cross-correlation between input signal and trigger photons, obtained by scanning the transverse position of the input signal; ( c ) cross-correlation function between retrieved signal and the trigger photons. The solid lines in ( b ) and ( c ) are theoretical fits. All data are raw, without noise. Full size image Figure 2 provides clear experimental evidence that an image memory at the true single-photon level can be realized using a cold atomic ensemble, the main features of the image had been preserved during storage. Moreover, the non-classical correlation between the trigger photon and the retrieved photon was retained. This point is crucial for establishing high-dimensional quantum repeaters. In this experiment, the main noise that reduced the signal-to-noise ratio was from the photon generated through the atomic transition of 5P 1/2 (F′=3)−>5S 1/2 (F=3). To eliminate this, we ensured the atomic population in state |2> was as near to zero before performing the storage experiment. This was achieved as follows: at the end of the trapping cycle and before the coupling laser was turned on, the atoms were pumped to state |1> by turning off the trapping laser 0.5 ms ahead of the repump laser. Dephasing between the two ground states induced by the Earth's magnetic field had an effect during storage, which shortened the storage time and reduced the storage efficiency. It is theoretically predicted that the efficiency of the EIT-based memory could approach unity in an atomic ensemble at a high OD [31] . In our experiment, the memory OD is about 10; therefore, we could improve the efficiency by increasing OD. The storage efficiency can be substantially improved by optimizing the pulse shape to match the EIT bandwidth [32] , [33] . We could make the single-photon wave packet match the memory bandwidth to increase the storage efficiency. In Chen et al . [29] , 78% storage efficiency is obtained via EIT in a cold atomic ensemble, where the techniques of matching the pulse shape to the EIT bandwidth and increasing OD of the atomic ensemble are applied. One main issue affecting the retrieved image quality was atomic diffusion, seen as softening at the edges of the image [13] , [22] . This problem can be solved using a 4-f imaging system that Fourier transforms the image that is then stored, instead of the image itself, in the atomic ensemble. Thus, diffusion can be reduced significantly [13] , [22] and the image can be stored for a much longer time. Storing a polarization state of a single photon To use our scheme in practice, we have to prove that photon coherence is preserved during storage. For this purpose, we performed two experiments. In the first, we experimentally checked whether we could store an arbitrary polarization state of the input signal photon. For that, we performed quantum-storage process tomography [34] , aided by a Sagnac interferometer ( Fig. 3a ). In this process, the two phase plates were removed from the interferometer. The whole setup consisted of the following three parts: state preparation of an arbitrary polarization state; Sagnac interferometry for storing the polarization state; and state tomography for state analysis. In this experiment, the photon did not carry a spatial structure. Using such a configuration, two orthogonal polarizations, either forward or backward directed, of an input state were stored in the atomic ensemble. The experimental details are presented in the Methods. 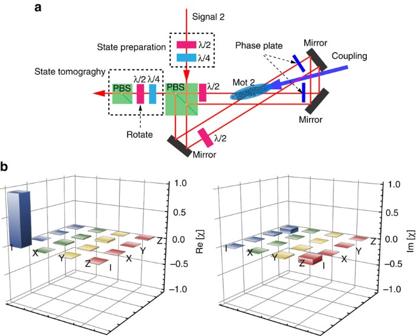Figure 3: Quantum process tomography of storing a polarization state of a true single photon. (a) Schematic of the simplified experimental setup demonstrating coherence of a single photon.λ/2(λ/4): a half-wave plate (a quarter-wave plate). PBS: Glan–Taylor polarization beam splitter with the extinction ratio of 105:1. (b) Calculated real and imaginary parts of the storage process matrixχobtained from experimental data in the Pauli operator basis {I,X,Y,Z}. For an ideal quantum memory device, theχmatrix should be peaked only at {I,I}. All data are raw, without noise correction. Figure 3b depicts the process matrix χ constructed according to experimental data. The calculated fidelities of the storage process were 0.94, 0.96, 0.98 and 0.96 for the four different input polarization states H , V , R and D , respectively, where H and V stand for horizontal and vertical polarizations, respectively, right-circular polarization, and diagonal polarization. In this process, the storage time was programmed for 100 ns. The experiment clearly demonstrates that photon coherence is preserved during storage. Using the Sagnac interferometer avoids phase fluctuations between the two orthogonal polarizations of the signal. Experimental details appear in the Methods. Figure 3: Quantum process tomography of storing a polarization state of a true single photon. ( a ) Schematic of the simplified experimental setup demonstrating coherence of a single photon. λ /2( λ /4): a half-wave plate (a quarter-wave plate). PBS: Glan–Taylor polarization beam splitter with the extinction ratio of 10 5 :1. ( b ) Calculated real and imaginary parts of the storage process matrix χ obtained from experimental data in the Pauli operator basis { I , X , Y , Z }. For an ideal quantum memory device, the χ matrix should be peaked only at { I , I }. All data are raw, without noise correction. Full size image Storing an OAM superposition state of a single photon In the second experiment, we verified whether we could store an OAM superposition state of the input signal photon. For that, we inserted the two phase plate (VPP-2, RPC Photonics) into the two optical paths (see Fig. 3a ) and the photon state of the input signal, with l =2 prepared for storage. The output state evolves into with a 45° rotation after the retrieved signal passes a quarter-wave plate. Next, a half-wave plate (see Fig. 3a ) rotates the photon polarization to yield the output state, where Û HWP ( θ ) is the transformational matrix of the half-wave plate with θ being the angle of the fast axis with respect to the vertical axis. The output state can be written as: Here interference between two terms in equation (3) gives rise to a characteristic pattern comprising four spots. Shifting the relative phase of the two terms causes this pattern to rotate. In our experiment, rotating the half-wave plate shifts the phase—that is changing θ continuously. In the actual experiment, we first used weak coherent light (~10 4 photons per pulse) as the input signal. We set the angle of the half-wave plate at θ =22.5°, 67.5°, 112.5° and 157.5°, respectively, and using a CCD camera (1,024 × 1,024, iStar 334T series, Andor) monitored the spatial shape of the light. The results given in Fig. 4a show that theoretical simulations and experimental data are in good accord. In addition, we focused the photons in a single spot into a fibre and detected these using a photon detector (Avalanche diode, PerkinElmer SPCM-AQR-15-FC). From equation (3), we know that and have an additional phase, and −2 θ , respectively. The detected intensity of the interference pattern will vary sinusoidally as sin(4 θ ) as the plate angle changes. In this experiment, we used the true single photon (signal 2 photon, generated through SFWM in MOT 1) as the input signal. Storage time was programmed at 100 ns. The integrated coincidence counts per second in a 50-ns coincidence window with background noise subtracted showed a clear interference pattern against plate angle ( Fig. 4b ) with a visibility of 0.74±0.1, the error being statistical arising mainly from noise from the coupling laser and the multiphoton events. Moreover, the experiment and the theory agreed well. The results presented clearly demonstrate that coherence between two different OAM photon states is preserved during storage. 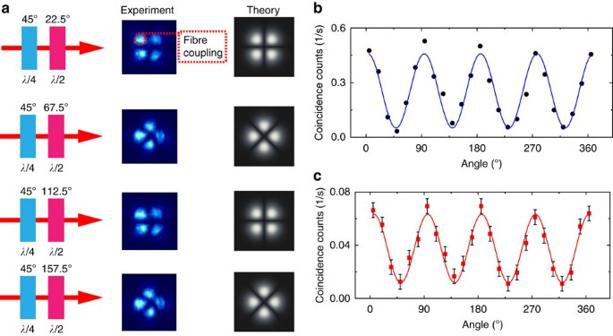Figure 4: Storing a superposition state of OAM. (a) Rotated interference patterns at different angle settings of the half-wave plate (seeSupplementary Movie 1).The left column represents the experimental angle settings of the half-wave and the quarter-wave plates. The middle column is the experimental results and the right column is the theoretical simulations; (b) interference pattern of the input signal photon as a function of plate angle; (c) interference of retrieved signal with plate angle. Blue and red lines are fits of the sinusoid sin(4θ). The background noise has been subtracted. Error bars represent±one standard deviation and are obtained based on the count statistics of single photons. Figure 4: Storing a superposition state of OAM. ( a ) Rotated interference patterns at different angle settings of the half-wave plate (see Supplementary Movie 1 ).The left column represents the experimental angle settings of the half-wave and the quarter-wave plates. The middle column is the experimental results and the right column is the theoretical simulations; ( b ) interference pattern of the input signal photon as a function of plate angle; ( c ) interference of retrieved signal with plate angle. Blue and red lines are fits of the sinusoid sin(4 θ ). The background noise has been subtracted. Error bars represent±one standard deviation and are obtained based on the count statistics of single photons. Full size image In this work, we provided the first evidence of the storage in a cold atomic ensemble of a true single-photon-carrying spatial structure. Although our work is a proof of principle, with a long way to go before being practical, it makes an important step towards realizing high-dimensional quantum memory. It accompanies recent progress in infrared-to-visible wavelength conversion [35] and long-distance fibre transmission of photons encoded in high-dimensional states [36] , as well as the significant advances in quantum key distribution transmission between ground and air [37] , [38] . All these results show that it is promising for establishing a high-dimensional quantum network in the future. Next, we will do some experiments related to the storage of a single-photon carrying higher OAM or a high-dimensional superposition state. We could also perform teleportation experiments using AOM states or perform the frequency conversion of single photons carrying AOM in the future. Experimental preparation of a true single photon A cigar-shaped atomic cloud of 85 Rb atoms obtained in MOT 1 (see Fig. 1a ) was used to prepare a real single photon via the SFWM in a double-lambda configuration, in which the states used were |1>, |2>, |3> and |4>, corresponding to energy levels 5S 1/2 (F=3), 5S 1/2 (F=2), 5P 3/2 (F′=1) and 5P 1/2 (F′=3), respectively. Pump 1 was from an external-cavity diode laser (DL100, Toptica), operating at wavelength 780 nm, and was set to be red-detuned at 50 MHz to the atomic transition of 5S 1/2 (F=3)−>5P 3/2 (F′=1). Pump 2, from another external-cavity diode laser (DL100, Toptica), operating at wavelength 795 nm, was set to resonate at the atomic transition 5S 1/2 (F=2)−>5P 1/2 (F′=3). Pumps 1 and 2 have opposite linear polarizations; signals 1 and 2 obtained through SFWM were also oppositely polarized. The power of pumps 1 and 2 were 54 μW and 0.65 mW, respectively. The OD of MOT 1 was about 8. Under phase-matching conditions and conversation of energy, the generated photons from signals 1 and 2 were non-classically correlated in the time domain. In the experiment, signal 1 and signal 2 photons were coupled into two single-mode fibres with a 90% coupling efficiency. Before that, an interference filter with a transmission coefficient of 50% was used to reduce the noise along the transmission path of signal 1. In addition, two home-made Fabry–Perot (FP) etalons were inserted into the optical paths of the signal 1 and the signal 2 photons to further reduce noise. Each FP had a transmission efficiency of 83% and a 500-MHz bandwidth. Subsequently, signal 1 photons were detected using a single-photon detector (Avalanche diode, PerkinElmer SPCM-AQR-15-FC with 50% efficiency), whereas signal 2 photons were stored for follow-up experiments. After having been stored for a specified time, the retrieved signal 2 photon was detected using another single-photon detector of the same make. The outputs from both detectors were connected to a time-to-digital converter (Fast Comtec. P7888) with 1 ns bin-width to measure the cross-correlation function g s1,s2 ( τ ). Usually classical light satisfied the following equation [26] : where g s1,s2 ( τ ), g s1,s1 (0) and g s2,s2 (0) were the normalized second-order cross-correlation and auto-correlation of the photons, respectively. The normalized g s1,s2 ( τ ) can be obtained by normalizing the true two-photon coincidence counts to the accidental two-photon coincidence counts g s1,s2 (∞). With τ = t s1 − t s2 , the relative time delay between paired photons, the maximum g s1,s2 ( τ ) we obtained in the experiment was g s1,s2 ( τ )=200±4 at τ =19 ns. Thus, the corresponding Cauchy–Schwarz inequality factor R =10,000±400 was much larger than 1 using the fact that g s1,s1 (0)= g s2,s2 (0)≈2 (photons from signals 1 and 2 exhibited photon statistics typical of thermal light). The Cauchy–Schwarz inequality is strongly violated, clearly demonstrating a non-classical correlation between photons. The full-width at half-maximum of the cross-correlation function was 32.5 ns; therefore, we estimated that the frequency full-bandwidth at half maximum of the photon was ~30 MHz. The photon bandwidth could be tuned, for example, by changing the Rabi frequency of the pump beam [39] . For an ideally prepared single-photon state, α tends to be zero, for a classical field, α ≥1, based on the Cauchy–Schwarz inequality [27] , [28] . A pure single photon has α =0 and a two-photon state has α =0.5. Therefore, α <1.0 violates the classical limit and α <0.5 suggests the near-single-photon character. Here the anticorrelation parameter was given by the ratio of various photoelectric detection probabilities, which were measured by the set of detectors D 1 , D 2 and D 3 . P 1 was the trigger photon counts, P 12 and P 13 were the twofold coincidence counts between the trigger and the two separated signal photon (the signal was divided into two equal parts by a beam splitter and detected by two single-photon detectors D 2 and D 3 , not shown in Fig. 1 ) and P 123 was the threefold coincidence counts between the three detectors D 1 , D 2 and D 3 . Experimental storage of a true single photon The experimental storage of a single photon through EIT was implemented in another MOT 2 ( Fig. 1b ). The OD of MOT 2 was about 10. The bandwidth for storage was about ~20 MHz. The coupling laser beam, from the same laser as the beam for pump 1, coupled the atomic transition of 5S 1/2 (F=2)−>5S 1/2 (F′=2). The signal photon produced is to be stored and the trigger is to be detected at detector 1. The output electrical signal from detector 1 was input to an arbitrary function generator (AFG 3252) to trigger an acousto-optic modulator to switch the coupling laser on and off with a rising–falling edge of 15 ns. The signal was first transmitted through 200 m of single-mode fibre and then was focused on the atomic cloud established in MOT 2 using a lens with a focal length of 500 mm. The coupling beam was focused using a 700-mm-focal-length lens, that covered the probe beam completely. The Rabi frequency of the coupling laser was 4 Γ , where Γ is decay rate of level .The angle between the coupling beam and probe was 3°. The non-collinear configuration used in the experiment significantly reduced noise from the coupling beam scattering. The retrieved signal was coupled into a single-mode fibre and was detected using another detector. We performed our experiment with a repeat rate of 100 Hz. The atomic trapping time was 8 ms, the experimental window was 1.5 ms and another 0.5 ms was used to prepare the initial state. Experimental quantum process tomography of a true single photon The experimental conditions of the quantum process tomography [34] of arbitrary polarizations were similar to the previous experiment, aside from the following: in regard to the photon-pair source based on SFWM, the power of pumps 1 and 2 were 120 μW and 1 mW, respectively. Pump 1 was set to red-detuned 170 MHz to the atomic transition of 5S 1/2 (F=3)−>5S 1/2 (F′=1). In the experiment, the coupling efficiency for the trigger and signal photons into two single-mode fibres was 85%. The previous interference filter was replaced by two new interference filters, with transmission efficiencies >95% at 780 nm. To reduce beam noise from pump 2 and the coupling laser, the previous FP etalon (inserted in the signal optical path) was replaced by two new FP etalons (one with transmission efficiency of 83%, another of 90%). The full bandwidth at half maximum of the photon was ~13 MHz. Concerning storage in the second MOT, the signal photon was focused into the second atomic cloud using a 1.9-m focal-length lens. The Rabi frequency of the coupling laser was 5 Γ. The coupling beam was an elliptical laser beam with size 1 × 3.5 mm in the atomic ensemble covering the probe beam completely. The retrieved signal photon was coupled with a single-mode optical fibre with the efficiency of 50%. We inserted two FP etalons to reduce noise from the coupling beam with an attenuation rate of ~50,000. How to cite this article: Ding, D.-S. et al . Single-photon-level quantum image memory based on cold atomic ensembles. Nat. Commun. 4:2527 doi: 10.1038/ncomms3527 (2013).